Mechanism of tetracycline resistance by ribosomal protection protein Tet(O) Tetracycline resistance protein Tet(O), which protects the bacterial ribosome from binding the antibiotic tetracycline, is a translational GTPase with significant similarity in both sequence and structure to the elongation factor EF-G. Here, we present an atomic model of the Tet(O)-bound 70S ribosome based on our cryo-electron microscopic reconstruction at 9.6-Å resolution. This atomic model allowed us to identify the Tet(O)-ribosome binding sites, which involve three characteristic loops in domain 4 of Tet(O). Replacements of the three amino-acid tips of these loops by a single glycine residue result in loss of Tet(O)-mediated tetracycline resistance. On the basis of these findings, the mechanism of Tet(O)-mediated tetracycline resistance can be explained in molecular detail. Tetracycline (Tc) is a broad-spectrum antibiotic active against both Gram-positive and Gram-negative bacteria, and used in a variety of medical and veterinary applications [1] . It targets the small subunit of the bacterial ribosome [2] , with the primary high-affinity binding site located beneath helix 34 of the 16S rRNA, in a crevice between the head and platform of the 30S subunit, in close vicinity of the A-site codon [2] . In this binding site, Tc partially occupies the space where an aminoacyl-tRNA would approach the A-site codon during the decoding process. Thus, Tc binding prevents any entering aminoacyl-tRNA from being recognized by the codon in the messenger RNA and thereby incapacitates the ribosome for protein synthesis [3] . Resistance to Tc is mediated through one of several mechanisms: Tc efflux, protection of the Tc binding site by binding of specific cytoplasmic proteins to the ribosome, Tc modification, or modification of 16S rRNA at the Tc-binding site [4] . These mechanisms are facilitated by over 20 different groups of tetracycline-resistance proteins [5] . Several of these proteins—the best-known being Tet(M) and Tet(O)—are paralogs of the translational GTPase EF-G [6] and actively remove Tc from the ribosome in a GTP-hydrolysis-dependent manner [7] , [8] . Detailed information on the Tet(O)-induced conformational changes of the ribosome to disrupt Tc binding is essential for understanding their mechanism of action. A previous Tet(O) cryo-electron microscopic (EM) study [9] , with a density map at a resolution of 16 Å, allowed the visualization of Tet(O) bound to the Escherichia coli ribosome, revealing that Tet(O) indeed has a similar shape as EF-G and binds to the same general site within the intersubunit cavity of the ribosome. Overall, the ribosomal complex was seen to closely resemble the conformation of the EF-G–70S ribosome complex stabilized with GDPNP. Sequence homology shows that Tet(O) shares the five structural domains with EF-G, the first two containing the GTP-binding site and being close to the GTP-associated centre of the 50S ribosomal subunit, whereas the other three domains are distinct for Tet(O) and are associated with its specific functions [9] , [10] . The high degree of sequence homology shared by Tet(O) and EF-G [11] makes it possible to build an atomic model of Tet(O) based on the X-ray structure of EF-G, using a cryo-EM map as constraint, provided its resolution is sufficient. The existing 16-Å reconstruction of Tet(O)-70S [9] is unsuitable for this purpose. In this study, we obtained an improved cryo-EM map of the E. coli 70S ribosome in complex with GDPNP-bound Tet(O) from Campylobacter jejuni , the best-characterized ribosomal protection protein, with a resolution of 9.6 Å. Guided by this higher-resolution map, a map-fitted atomic model of the ribosome-Tet(O) complex has allowed us to determine the binding sites between Tet(O) and the ribosome. Our results indicate that the critical residues of Tet(O) would clash with Tc if both were present in the same ribosome complex; thus the presence of Tet(O) is poised to disrupt the binding of Tc. These critical residues are located in three loops of domain 4, whose positions with respect to the ribosome are different than for EF-G [12] . Moreover, our structural results are strongly corroborated by our mutational and biochemical data. Multiple tests of the three Tet(O)’s loops with either a single Ala mutation in one of the three loops, or a replacement of any of the three residues tipping the three loops by a glycine, resulted in loss of Tet(O) functionality as measured by minimum inhibitory concentration (MIC) of the antibiotic resistance of E. coli strains. Together, these results allow us to understand the structural basis for the Tc resistance mechanism on the molecular level. Cryo-EM density map of Tet(O) bound with the 70S ribosome We obtained a three-dimensional cryo-EM density map for the complex of Tet(O) bound with the 70S ribosome in the presence of the nonhydrolyzable GTP analogue GDPNP at a resolution of 9.6 Å (FSC=0.5 criterion, Supplementary Fig. S1 ). The map was reconstructed using the single-particle reconstruction approach along with image classification using a maximum-likelihood method (ML3D [13] ) as well as supervised classification. The classification results indicate a very high (more than 90%) occupancy of Tet(O) in the complex with the 70S ribosome. The density for Tet(O) in this improved map is at a position which agrees with that described in the earlier study [9] , but boundary and shape are better defined in the context with the 70S ribosome ( Fig. 1 ). 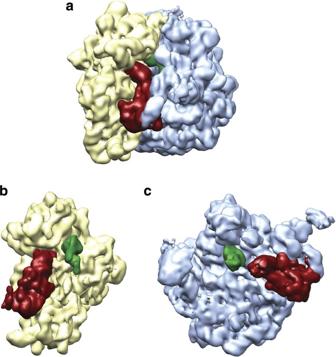Figure 1: Cryo-EM maps of the 70S ribosome fromE. colibound with Tet(O). (a) 70S·Tet(O)·GDPNP·fMet-tRNA complex. The map is segmented to show the 30S subunit (yellow), the 50S subunit (blue), Tet(O) (red) and the P-site tRNA (green). The same colour scheme is used for panelsa–c. (b) Density for the 30S subunit with Tet(O) and P-site tRNA. (c) Density for the 50S subunit with Tet(O) and P-site tRNA. Figure 1: Cryo-EM maps of the 70S ribosome from E. coli bound with Tet(O). ( a ) 70S·Tet(O)·GDPNP·fMet-tRNA complex. The map is segmented to show the 30S subunit (yellow), the 50S subunit (blue), Tet(O) (red) and the P-site tRNA (green). The same colour scheme is used for panels a – c . ( b ) Density for the 30S subunit with Tet(O) and P-site tRNA. ( c ) Density for the 50S subunit with Tet(O) and P-site tRNA. Full size image To date, Tet(O)’s structure has not been solved by crystallography. In the present study, the improved resolution of the density map allowed us to build an atomic model of Tet(O), guided by its homology to EF-G, and characterize its binding interactions with the ribosome. First, a sequence alignment of C. jejuni Tet(O) and Thermus thermophilus EF-G was created, guided by the crystal structure of EF-G (PDB accession code: 2WRI ) using the 3D-coffee software [14] To compare site-specific sequence conservation across the entire Tet(O) and EF-G families, a data set of sequences belonging to both of these families was assembled. Tet(O) sequence homologues, representing the Tet family of translational GTPases (trGTPases), were retrieved from the NCBI using BlastP. These sequences were aligned with a data set of previously identified sequences from the EF-G family [15] , and consensus sequences were generated for each family. The sequence alignment results indicate a high sequence similarity (50%) between Tet(O) and EF-G, a firm basis for using homology modelling ( Supplementary Fig. S2 ). In all these sequences, the highly conserved nucleotide-binding motifs are perfectly aligned, and the sequence of Tet(O) is divided into five domains, corresponding to the domains defined by the sequence of EF-G. The alignment of C. jejuni Tet(O) and T. thermophilus EF-G was used to create a homology model of Tet(O) using the program Modeller [16] . Our model of Tet(O) closely resembles the structural features of EF-G, which is in a 70S ribosome-bound GTP form ( Fig. 2 ). The Tet(O) model together with the X-ray structure of the 70S ribosome [17] was fitted into the entire cryo-EM map for the complex using the Molecular Dynamics Flexible Fitting method [18] . The fitted structure, as shown in Fig. 3 , closely captures the conformation of the entire complex as formed in the density map, which allows us to characterize the interactions between Tet(O) and the ribosome in detail. We validated the fitting structure by using a different crystal structure of the 70S ribosome as the starting structure for the molecular dynamics flexible fitting (MDFF; 2WRI, 2WIJ). The resultant structure of Tet(O) as well as the bases rearrangement in the 16S rRNA are in good agreement with the model presented in the manuscripts. The root-mean-square deviation of the two 70S ribosomal structures is just 1.5 Å, and just 1.7 Å for all atoms of Tet(O). 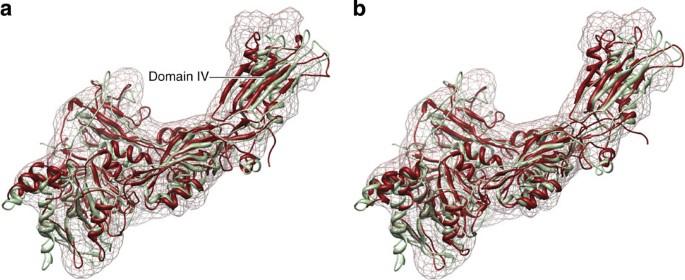Figure 2: Homology model of Tet(O). (a) The initial Tet(O) model (red) and the EF-G structure (green, PDB code: 2WRI) are shown as overlaid ribbons in the segmented density map (red mesh). The three loops in domain IV are seen to be positioned differently in the two structures. (b) The map-fitted structure of Tet(O) (red) is superimposed with the crystal structure of EF-G, showing the adjustment in the orientations of the three loops of Tet(O) into the density through the map fitting process. Figure 2: Homology model of Tet(O). ( a ) The initial Tet(O) model (red) and the EF-G structure (green, PDB code: 2WRI) are shown as overlaid ribbons in the segmented density map (red mesh). The three loops in domain IV are seen to be positioned differently in the two structures. ( b ) The map-fitted structure of Tet(O) (red) is superimposed with the crystal structure of EF-G, showing the adjustment in the orientations of the three loops of Tet(O) into the density through the map fitting process. 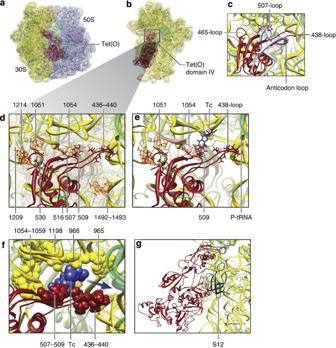Figure 3: Cryo-EM map-fitted atomic model of the 70S ribosome bound with Tet(O). (a) Cryo-EM map, displayed as transparent mesh, with atomic model displayed as ribbons. The 16S rRNA is in yellow, proteins in the 30S subunit in green, 5S and 23S rRNA in blue, and proteins in the 50S subunit in pink. Tet(O) is in red, P-site tRNA in dark green. (b) The 30S subunit with Tet(O) and P-site tRNA shown inais displayed after a clockwise rotation around vertical (in plane) axis by 90°, to show the interface with the 50S subunit. (c) Tet(O)’s domain IV (red), superimposed with the anticodon stem and loop of an A/T-site tRNA (grey) in the decoding region of the 30S subunit. The overlap between Tet(O) and the tRNA occurs at the 507- and 438-loops. (d) Zoomed-in view of the area marked by green box inb. (e) Portion of the 16S rRNA (pink) surrounding Tc, superimposed on the 16S rRNA (yellow) in the current Tet(O)-bound model. The 507-loop is seen to clash with the site for Tc (blue). Nucleotides 1051 and 1054 in the 16S rRNA are seen to be reoriented in the two structures. (f) The 507-loop, 438-loop and a portion of the 30S subunit including nucleotides 966, 1196 and their surrounding nts form a structural corridor for a possible release of Tc. (g) Tet(O)-S12 contact sites. S12 is shown in dark green. Full size image Figure 3: Cryo-EM map-fitted atomic model of the 70S ribosome bound with Tet(O). ( a ) Cryo-EM map, displayed as transparent mesh, with atomic model displayed as ribbons. The 16S rRNA is in yellow, proteins in the 30S subunit in green, 5S and 23S rRNA in blue, and proteins in the 50S subunit in pink. Tet(O) is in red, P-site tRNA in dark green. ( b ) The 30S subunit with Tet(O) and P-site tRNA shown in a is displayed after a clockwise rotation around vertical (in plane) axis by 90°, to show the interface with the 50S subunit. ( c ) Tet(O)’s domain IV (red), superimposed with the anticodon stem and loop of an A/T-site tRNA (grey) in the decoding region of the 30S subunit. The overlap between Tet(O) and the tRNA occurs at the 507- and 438-loops. ( d ) Zoomed-in view of the area marked by green box in b . ( e ) Portion of the 16S rRNA (pink) surrounding Tc, superimposed on the 16S rRNA (yellow) in the current Tet(O)-bound model. The 507-loop is seen to clash with the site for Tc (blue). Nucleotides 1051 and 1054 in the 16S rRNA are seen to be reoriented in the two structures. ( f ) The 507-loop, 438-loop and a portion of the 30S subunit including nucleotides 966, 1196 and their surrounding nts form a structural corridor for a possible release of Tc. ( g ) Tet(O)-S12 contact sites. S12 is shown in dark green. Full size image Interactions between Tet(O) and the ribosomal 30S subunit Tet(O) binds with the ribosome on both the 30S and 50S subunits. On the 30S subunit, the three loops in domain IV of Tet(O), namely the 465-, 507- and the 438-loop, insert into the head-platform crevice, spanning across about 30 Å ( Fig. 3c ). The large spatial expansion of the three loops may allow them to have various roles in their binding with the ribosome, in jointly conveying Tc resistance. The 507-loop and the 438-loop occupy approximately the position where the anticodon stem–loop of an A-site tRNA would occur in a normal translating ribosome, while the 465-loop extends into the structural pocket formed between nucleotides 1055 and 1209 within helix 34 ( Fig. 3c ). Although this third loop is placed outside the decoding centre at the A-site, it apparently has a role in restraining the structural flexibility between the 1055 and 1029 ends. The 507-loop, which is located in the middle of the lined-up three loops, appears to have the most direct, and most crucial role in bestowing tetracycline resistance as evident from its position relative to Tc. The position of Tc in the 30S subunit, as revealed by the crystallographic study [2] , was mapped to the current structure of the 30S subunit ( Fig. 3e ). This position would result in a spatial clash between residues 507–509 and Tc if both were present in the same complex, that is, either Tc or the Tet(O)’s 507-loop would exclusively occupy the same space. Unlike the 507-loop, the 438-loop is not involved in the interactions with Tc, located about 15 Å away from Tc, but residue 437 is located in the near vicinity of nucleotides 1492–1493 in the 16S rRNA, where the decoding interaction network is observed in a normal translation ribosome [19] . We observe that this loop and nucleotides around 966 and 1196 of the 16S rRNA with their surrounding nucleotides form a corridor, which starts at the position of Tc and leads to the outside of the ribosome ( Fig. 3f ). The dissociating Tc molecule has to navigate this corridor, which acts as the only pathway for the molecule’s release from the ribosome, which might explain the high activation energy of the process [8] . The presence of the 465-loop inside the structural pocket near nucleotides 1051 and 1209 in the 16S rRNA leads to a local distortion of the 16S rRNA, in the immediate vicinity of the Tc-binding site ( Fig. 3d ). According to the Tc-bound 30S subunit, this loop occupies the position of nt 1209. The presence of the 465-loop of Tet(O) at the base of the 30S subunit’s beak prevents the head of the 30S subunit from rotating, a motion required in the normal course of mRNA–tRNA translocation [9] . Tet(O) interacts with the 30S subunit protein S12 closely at domain III, and possibly at domain IV of Tet(O) ( Fig. 3g ). Residues 358 and 379 in domain III of TetO seem to be directly to interact with S12’s residues 74–76. The S12 residues 483 and 517 are located at the base of the 507- and 465-loops of Tet(O), respectively. This interaction between S12 and Tet(O) at multiple sites is similar to the bridge-like connexion that S12 forms with two sites of the A/T-site tRNA in the EF-Tu–tRNA complex, as previously described for the X-ray structure of the ternary complex-bound ribosome complex [20] . It is worth noting that the Tet(O) 438-loop is located close to the mRNA around the A-site codon, as shown in our map-fitted structure. The point of closest approach (within 3 Å) occurs between residue 438 and the second nucleotide for the A-site codon. Functional importance of Tet(O) domain 4 loops Independently from the structural study, we carried out multiple mutation and substitution experiments on the three loops of Tet(O) identified in the atomic model. To determine the mutation sites and the substitution sites, we started with a comparison of the sequence conservation of Tet-like proteins and EF-G proteins in domain 4. Tet(O) sequence homologues, representing the Tet family of trGTPases, were retrieved from the NCBI using BlastP. These were aligned with a data set of previously identified sequences from the EF-G family [15] , and consensus sequences were generated for each family. The alignment shows that the Tc-interacting loops are differentially conserved between EF-G and Tet families, particularly in the 438- and 507-loop, which have very different amino-acid compositions. However, these loops are not very strongly conserved within the entire Tet family; only 2 out of 6, 6 out of 11 and 4 out of 8 residues are conserved at >60% in the 438-, 465- and 507-loops, respectively ( Fig. 4a ). This suggests that a certain amount of sequence variation is tolerated in the loops, while functionality is maintained. 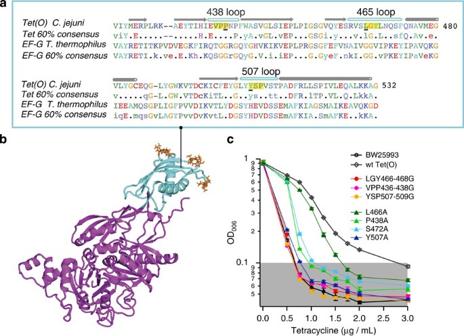Figure 4: The involvement of Tet(O) loops in Tc resistence. (a) Alignment ofC. jejuniTet(O) (NCBI GI number 51209514),T. thermophilusEF-G (NCBI GI number 46199633) and consensus sequences of domain 4 from the Tet(O) and EF-G families. In the consensus sequences, a residue is capitalized if it present for more than 60% of the time in the full alignment; a lowercase letter shows 60% conservation within a common substitution group, and a dot shows a position that does not meet either of these thresholds. The secondary structure is indicated above the alignment with arrows for β-strands, with the functionally important loops at the tip of the domain labelled. The sites of point mutations in Tet(O) are indicated by underlining, and three amino-acid deletions by yellow highlighting. (b) Full-length Tet(O) homology model structure with domain 4 rendered in teal. Residues rendered in orange sticks are those subjected to mutational analysis, as shown inaandc. (c) Tetracycline sensitivity measurements. The optical density at 600 nm after 12 h of bacterial growth at 37 °C is plotted as a function of tetracycline concentration. The error bars represent standard deviations, and each experiment was performed at least three times. Tetracycline concentration at which OD600was below 0.1 was treated as the MIC. Figure 4: The involvement of Tet(O) loops in Tc resistence. ( a ) Alignment of C. jejuni Tet(O) (NCBI GI number 51209514), T. thermophilus EF-G (NCBI GI number 46199633) and consensus sequences of domain 4 from the Tet(O) and EF-G families. In the consensus sequences, a residue is capitalized if it present for more than 60% of the time in the full alignment; a lowercase letter shows 60% conservation within a common substitution group, and a dot shows a position that does not meet either of these thresholds. The secondary structure is indicated above the alignment with arrows for β-strands, with the functionally important loops at the tip of the domain labelled. The sites of point mutations in Tet(O) are indicated by underlining, and three amino-acid deletions by yellow highlighting. ( b ) Full-length Tet(O) homology model structure with domain 4 rendered in teal. Residues rendered in orange sticks are those subjected to mutational analysis, as shown in a and c . ( c ) Tetracycline sensitivity measurements. The optical density at 600 nm after 12 h of bacterial growth at 37 °C is plotted as a function of tetracycline concentration. The error bars represent standard deviations, and each experiment was performed at least three times. Tetracycline concentration at which OD 600 was below 0.1 was treated as the MIC. Full size image We validated our structural results by testing the effects of mutations of Tc-interacting regions on Tet(O) functionality in vivo , as judged by measuring the antibiotic resistance of E. coli strains transformed with plasmid-expressed Tet(O) mutants ( Fig. 4c ; Table 1 ; Supplementary Table S1 ). These mutations and deletions were targeted in the three characteristic loops in domain 4 of Tet(O), at those residues that are either directly or closely involved in the interactions in the Tc-binding site. The effects of the mutations and deletions on Tet(O) functionality were measured through the reduction in the MIC in each case. As a reference we used BW25993 E. coli strain transformed with a plasmid-expressed wild-type Tet(O), with a Tc MIC of 2 μg ml −1 and untransformed BW25993 E. coli , MIC 0.5 μg ml −1 . Table 1 Functional characterization of Tet(O) variants mutated in Tc-interacting loops. Full size table First, we tested the 507-loop, which is positioned to directly compete with Tc. Replacement YSP507-509G resulted in complete loss of Tet(O) activity, whereas mutation Y507A resulted in 83% loss of Tet(O) activity. These results indicate crucial importance of the 507-loop for the Tet(O)’s ability to protect the ribosome from Tc. These results agree with the structural model based on our cryo-EM study, as well as an earlier mutational study of the 507-loop [10] . Second, we examined the involvement of the 465-loop, which is oriented in the vicinity of the Tc-binding site as shown in the atomic model. A point mutation of the two sites, L466A or S472A, resulted in a 33% and 76% inhibition of Tet(O)-mediated resistance, respectively. However, substitution of residues 466–468 by a single glycine (LGY466-468G) resulted in complete inhibition of Tet(O) activity. These results suggest that the residues in the 465-loop collectively have an important role in the Tet(O)’s function, even though sequence variation is tolerated in the loops, again as predicted from the position of this loop in the model and the conservation analysis. Finally, we checked the functional role played by the 438-loop, which is positioned outside the binding vicinity of Tc. A single-point mutation (P438A) and substitution of the three residues 436–438 by a glycine resulted in 83% and 100% inhibition, respectively. These results, combined with our structural data, verify the importance of our proposed corridor for Tc’s release from the ribosome (see Discussion). In summary, these results demonstrate that the integrity of the residues identified in our cryo-EM reconstruction as binding sites is crucial for Tet(O) functionality. The mutation results are fully consistent with our cryo-EM structural analysis. Interactions between Tet(O) and the ribosomal 50S subunit On the 50S subunit side, Tet(O) contacts the GTPase-associated centre, between residues 619–620 in domain III and nucleotides 1066 in helix 43 of the 23S rRNA. The residues of Tet(O) responsible for GTP hydrolysis form a similar structural pocket as in EF-G, which surrounds the sarcin-ricin loop (nts in the 2662-loop). It is in this pocket where the hydrolysis takes place. In the Tet(O) complex, the closest distance is found to be between nucleotide 2663 and residue 40, about 4 Å. The current map-fitted structure would need to be slightly adjusted around the GDPNP-binding position if GDPNP was included in the fitted structure. Interestingly, helix 69 of the 23S rRNA, which was repeatedly found to be involved in the interactions with other ribosomal factors such as the EF-Tu–aminoacyl-tRNA complex and EF-G [12] , [20] , is positioned beyond a bonding distance from Tet(O). The closest point (nucleotide 1914) is about 6 Å away from Tet(O). Therefore, in the current Tet(O)–ribosome complex, helix 69 has no direct involvement. Tet(O) binding-induced conformational changes in 30S The overall ribosome conformation displays no intersubunit rotation when Tet(O) is stalled on the ribosome in the presence of GDPNP. Essentially, binding with GDPNP allows Tet(O) to remain in its GTP form. This ribosome conformation agrees with the X-ray structure of the 70S ribosome bound with EF-G-GDP-fusidic acid [12] . However, a notable change of ribosomal conformation occurs in—a rearrangement that was identified using chemical footprinting [21] . In the complex with Tet(O), the backbone shape of helix 34 deviates from the normal structure as formed in the X-ray structures of the 30S subunit either bound or unbound with Tc ( Fig. 3e ). This RNA fragment in helix 34 includes a single-nucleotide bulge at 1051, as well as two unpaired nucleotides 1054–1055, and connects the rest of helix 34 on the two ends. These unpaired nucleotides naturally provide structural flexibility, which is evidently exploited in the binding of Tet(O) to the ribosome. Our structure shows that residue 507 in domain IV and nucleotide 1054 in helix 34 would spatially clash if the fragment of helix 34 remained in its normal position. Therefore, the binding of Tet(O) clearly causes a change in that region of backbone. Following the positional change in nucleotide 1209, the backbone shape of the fragment around nt 1051 also must adjust. The base of nucleotide 1054 in particular seems to have a crucial role in holding tetracycline on the ribosome based on the crystal structure by Gao et al. [12] (PDB ID 1HNW). Tetracycline adheres to the 30S subunit through multiple hydrogen bonds with nucleotide 1054. The position of nt 1054 in the current structure is reoriented from being in the Tc-bound ribosome, otherwise it would clash with the 507-loop in Tet(O). Another Tet(O) binding-induced change in the ribosome occurs at helix 18, including nucleotide 530, which is crucially involved in the network of bases during the normal decoding process. The Tet(O) residue 512–513 in the map-fitted structure are within bonding distance from nucleotides 516–519 of helix 18. This clash is resolved by the reorientation of nucleotide 516, which appears in a twisted conformation of helix 18 in our map-fitted structure. In this unusual conformation of helix 18, its nucleotide 530 is also reoriented. Evidently, the original orientation must be restored if translation on the ribosome were to resume after the Tet(O) is released from the ribosome along with Tc. The correction would have to be spontaneous after Tet(O) release. This subsequent untwisting process, which we must assume as part of the bacterial rescue of the ribosome, indicates a substantial flexibility of the structure of helix 18. In addition, the bases of nts 1492–1493 in the 16S rRNA flip out towards the Tet(O)’s 438-loop ( Fig. 3 ); the flipped-out conformation that was also observed when a codon–anticodon recognition takes place in a translating ribosome [19] . In this study, the structure of the 70S–Tet(O) complex in the presence of GDPNP has allowed us to visualize the details of binding between the 70S ribosome and Tet(O). In the GDPNP-bound form Tet(O) was earlier shown biochemically to promote release of Tc from the 70S ribosome [21] , [22] , and the elucidation of the current structure therefore provides direct functional insights into the mechanisms of Tet(O)-mediated Tc resistance. On the 30S subunit side, Tet(O) is positioned close to the site where Tc has been found in the X-ray structure. The 30S subunit-Tet(O) contact sites we have identified in the present study can be divided into two categories: (1) those which lead to a clash with the space for the binding of Tc via the 507-loop and (2) those which disrupt the structure of the 16S rRNA around the Tc-binding site via the 465-loop towards nucleotide 1209 in 16S rRNA. As in EF-G, the GTP-binding site in Tet(O) is located at the GTPase-associated centre. These contacts between the Tet(O) and the ribosome seem to collectively have the role of preventing or reversing the binding of Tc to the ribosome. The most direct effect of Tet(O) binding in preventing Tc from binding to the 30S subunit seems to be the result of a competition between residues 507–509 of Tet(O) and Tc for the same space. When Tet(O) enters into the Tc-bound ribosome, the 507-loop cannot be settled into the ribosome complex because Tc already occupies the close vicinity of nucleotide 1054 and forms multiple hydrogen bonds with the ribosome. The competition for the same site guarantees that Tet(O) and Tc cannot coexist in the ribosomal complex. In addition, binding of Tet(O) disrupts the ribosome structure and reshapes the geometry of the backbone where Tc is anchored ( Fig. 3e ). With this disrupted backbone structure, the nucleotides involved in binding with Tc are reoriented, and thus, Tc loses its bonds with the ribosome. Interestingly, the binding of Tc does not change the backbone shape from its shape in the Tc-free ribosome. The question arises is by which molecular mechanism Tc inhibits normal translation in the ribosome. One may ask why a Tc-bound ribosome does not accept an entering EF-Tu-bound aminoacyl-tRNA complex, but does accept Tet(O) even though the EF-Tu–aminoacyl-tRNA complex forms a shape highly similar to that of Tet(O). Our current study provides some insights to answer this question. If an aminoacyl-tRNA bound with EF-Tu enters into the ribosome, its anticodon loop must reach the codon site. In the presence of Tc, a primary portion of the space for the anticodon loop is already occupied by Tc ( Fig. 3e ), which causes a decisive rejection of the aminoacyl-tRNA from the ribosome before codon–anticodon recognition can take place. In contrast, Tet(O) enters the ribosome with less demand for space in that region than the anticodon loop of the tRNA; the available space provides an opportunity for Tet(O) to be admitted to the factor binding site, important for subsequence GTP hydrolysis. Tet(O), a GTPase, possesses a structure very similar to that of ribosomal GTPase, elongation factor G. The structural similarity suggests an analogy of their GTP-hydrolysis-induced conformational changes, which enable the two ribosomal proteins to perform their respective biological functions. The structural effects of the EF-G-associated GTP hydrolysis on the ribosome have been extensively studied [23] , [24] , [25] . It is known that GTP hydrolysis induces substantial conformational changes in the ribosome. The ribosome’s effect on the conformation of EF-G is substantial, as well, causing domain IV to be reoriented relative to the other domains, as shown by cryo-EM [24] and X-ray structures [12] of the ribosome bound with EF-G in the presence of fusidic acid. The antibiotic fusidic acid traps EF-G in a conformational intermediate between the GTP and GDP forms. In this translocational complex, a contact observed between the 507-loop of EF-G and the P-site tRNA seems to be essential for the translocation of tRNA based on the significant conformational flexibility of this loop [12] . This flexibility allows the loop to participate in the major dynamic motion of the entire domain IV as the GTP hydrolysis takes place. Thus, we see this loop as a functionally required structural element in EF-G. The structural similarity of Tet(O) to EF-G suggests structural flexibility in the equivalently positioned loops of Tet(O). Accordingly, we predict that GTP hydrolysis in Tet(O) results in extensive conformational changes in the distal loops of domain IV, particularly in the three flexible loops. By combining structural and mutational analyses, the present study provides structural insights into how the three loops in domain IV (see Fig. 3 ) might cooperate to expel Tc from the ribosome: the 465-loop is responsible for distorting the backbone shape at nucleotides 1051–1054 of 16S rRNA, which weakens or abolishes the binding of Tc at this site with the RNA; the 507-loop in the middle of these three directly pushes Tc out of the ribosome; and the 438-loop along with nucleotide 966 and 1196 should form a corridor allowing Tc to exit. After completion of this work, a cryo-EM reconstruction of a 70S–Tet(M) complex was published [26] . Our results agree with the results by Wilson and coworkers in all essential details, as expected based on the high sequence homology between Tet(O) and Tet(M). Sample preparation and image processing of ternary complexes The Tet(O)-ribosome complex was prepared using in vitro translation systems in polymix and HiFi buffers, respectively [27] , [28] . C. jejuni Tet(O) protein was overexpressed and purified as described previously [29] . To prepare samples for cryo-EM, aliquots of the ribosomal complexes were thawed separately on ice and diluted into the buffer to 40 nM concentration of ribosome, 4 μM Tet(O) and 400 μM GDPNP. Quantifoil 2/4 grids were used for cryo-EM and prepared following standard procedures [30] . The automated acquisition program AutoEMation [31] was used to collect CCD (charge-coupled device) images on an FEI Tecnai Polara at 200 kV and a nominal magnification of × 50,000. The microscope is equipped with a single-port 4K × 4K CCD camera (TVIPS TemCam-F415), corresponding to a pixel size of 2.71 Å. 1200 CCD images were selected which yielded about 110,000 particles using the SPIDER lfc pick procedure, and manually verification selected about 90,000 particles from these initial picks. The reconstruction procedure followed the reference-based projection-matching technique, which is implemented in the SPIDER program [32] , with 15 rounds of refinement and a final angular spacing of 1°. The particles were divided into 34 defocus groups, resulting in an initial reconstruction at a resolution of 12 Å. The map resolution was improved through the following classification process. The particles were classified using both unsupervised (using the ML3D program [13] ) and supervised classification approaches. ML3D, with either four or five classes settings, produced consistent density for the 70S-Tet(O) complex in all but one of the classes, in which about 10% of the total population showed the 50S subunit instead. This particle distribution was confirmed using supervised classification approach. Thus, the 10% non-70S ribosome particles were excluded from the final reconstruction. The final resolution for the map, after 15 rounds of angular refinement and a final angular spacing of 1°, was 9.6 Å, using a cutoff of 0.5 in the Fourier Shell Correlation. Sequence alignment and modelling of Tet(O) For assessing similarity between and among the EF-G and Tet(O) families of GTPases, 313 Tet(O) sequences were retrieved from the NCBI RefSeq database using BlastP with C. jejuni Tet(O) as the query. 171 EF-G sequences were taken from the data set of [15] and EF-G and TetO sequences were aligned with Mafft [33] . Consensus sequences were calculated with Consensus Finder [15] . To visualize a subset of aligned representative sequences from across the diversity of the Tet family, phylogenetic analysis was carried out using FastTree [34] (data not shown). For homology modelling, an alignment of TetO with EF-G was made with 3Dcoffee [14] , taking into account the structure of Thermus thermophilis EF-G (PDB ID 2WRI) [35] for the placement of insertions and deletions. The sequence alignment result was used to build an atomic model of Tet(O) using Modeller [16] . This atomic model and the X-ray structure of a 70S ribosome including a P-site tRNA [17] (PDB codes: 2J00, 2J01) were together fitted into the cryo-EM map by means of MDFF [18] , assuming a generalized-Born implicit solvent as implemented in NAMD [36] . Mutational validation of Tc-interacting regions of Tet(O) To measure the minimal inhibitory concentration (MIC) we used the Tet(O) plasmid, described in [19] , transformed into BW25993 E. coli . MICs were measured in 96-well plate format according to ref. 37 . Mutant versions of Tet(O) were constructed using the overlap extension PCR method [38] , [39] and KOD Hot Start DNA Polymerase (Novagen). Two complementary mutagenic primers (for generating substitution mutants) or two chimeric primers (for producing deletion mutants) were employed along with two flanking primers containing a Mun I restriction site. The amplified full-length mutant DNA was cut with Mun I, ligated into circular molecule and then transformed into DH5α cells. Resulting mutations were confirmed by sequencing. Accession codes: Electron microscopy density maps and coordinates have been deposited in EMDB under accession code EMD-26598. How to cite this article: Li, W. et al. Mechanism of tetracycline resistance by ribosomal protection protein Tet(O). Nat. Commun. 4:1477 doi: 10.1038/ncomms2470 (2013).